GIV/Girdin is a central hub for profibrogenic signalling networks during liver fibrosis Progressive liver fibrosis is characterized by the deposition of collagen by activated hepatic stellate cells (HSCs). Activation of HSCs is a multiple receptor-driven process in which profibrotic signals are enhanced and antifibrotic pathways are suppressed. Here we report the discovery of a signalling platform comprising G protein subunit, Gαi and GIV, its guanine exchange factor (GEF), which serves as a central hub within the fibrogenic signalling network initiated by diverse classes of receptors. GIV is expressed in the liver after fibrogenic injury and is required for HSC activation. Once expressed, GIV enhances the profibrotic (PI3K-Akt-FoxO1 and TGFβ-SMAD) and inhibits the antifibrotic (cAMP-PKA-pCREB) pathways to skew the signalling network in favour of fibrosis, all via activation of Gαi. We also provide evidence that GIV may serve as a biomarker for progression of fibrosis after liver injury and a therapeutic target for arresting and/or reversing HSC activation during liver fibrosis. Liver fibrosis is the consequence of an excessive deposition of collagen resulting from an imbalance between its synthesis and degradation. Upon liver injury, hepatic stellate cells (HSCs), the major collagen-synthesizing cells in the liver, become activated and transdifferentiate into myofibroblast-like cells that proliferate faster and display enhanced chemotaxis, survival and collagen production [1] . Such transdifferentiation is triggered by the activation of a diverse classes of receptors, for example, platelet-derived growth factor receptor (PDGFR) [2] , transforming growth factor β receptor (TGFβR) [3] , epidermal growth factor receptor (EGFR) [4] , vascular endothelial growth factor receptor (VEGFR) [5] , insulin/insulin-like growth factor receptor (IR/IGF1R) [6] , Gi-coupled chemokine/cytokine receptors (CCRs) [7] and Toll-like receptor 4 (TLR4) [8] , and two of them (TGFβR and PDGFR) have been widely studied and established as major profibrogenic receptors [2] , [3] . Regardless of the type of receptor activated, two key profibrotic signals, the PI3K-Akt and the SMAD signalling cascades [9] , must be enhanced to initiate and propagate HSC activation and collagen synthesis. Once activated, the PI3K-Akt pathway triggers fibrogenesis via three mechanisms—(1) by inactivating Forkhead box protein O1 (FoxO1), an antifibrotic transcription factor that suppresses transdifferentiation and proliferation of HSCs [10] , (2) by suppressing apoptosis [11] and (3) by further enhancing the TGFβ-SMAD-collagen pathway [11] . Although widely recognized as a key profibrotic trigger, the precise multireceptor-mediated mechanism(s) that drives unrestricted enhancement of the PI3K-Akt pathway remains elusive. Profibrotic pathways are antagonistically balanced by cyclic adenosine monophosphate (cAMP), a well-known and conserved antifibrotic signalling second messenger of G protein signalling cascades [12] . Accumulation of cAMP in HSCs is known to inhibit chemotaxis, proliferation and collagen synthesis, while simultaneously increasing the removal of collagen by metalloproteases [13] . Mechanistically, cAMP inhibits TGFβ-SMAD signalling at a transcriptional level via modulation of the protein kinase A (PKA)-cAMP response element-binding protein (CREB)-dependent pathway [14] . Although recognized as a key antifibrotic signal, the mechanism(s) by which cAMP levels are suppressed by multiple receptors during liver fibrosis remains unknown. We recently established that GIV, aka Gα-Interacting Vesicle-associated protein, is a multimodular signal transducer and a guanine nucleotide exchange factor (GEF) for trimeric Gi that modulates the key signalling events downstream of diverse classes of receptors, for example, growth factor receptor tyrosine kinases (RTKs), such as EGFR, IGF1R, VEGFR and InsR [15] , [16] , [17] , [18] and chemotactic G protein-coupled receptors (GPCRs) such as LPAR1 (refs 16 , 19 , 20 ). Working downstream of both RTKs and GPCRs, GIV serves as a common platform that enhances PI3K-Akt signals and reduces cAMP production, all via activation of Gi [16] . GIV modulates signalling during diverse biological processes including epithelial wound healing, macrophage chemotaxis, development, autophagy, angiogenesis, vascular repair and tumour metastasis (reviewed in ref. 21 ). As signalling pathways modulated by GIV are also the major components of the fibrogenic network, here we investigated whether GIV plays a role in the activation of HSCs during liver fibrosis. We found that GIV triggers HSC activation by coordinately reshaping the fibrogenic signalling network (enhances pro- and inhibits antifibrogenic signals) downstream of multiple receptors, all via activation of Gαi. As the fundamental signalling pathways driven by GIV are common to fibrogenic diseases afflicting other organs, insights gained will have an impact on the understanding, approach and the paradigms of diverse fibrosis-related diseases. GIV is upregulated in the liver after fibrotic injury We previously showed that expression of GIV is upregulated during epithelial wound healing [22] . As liver fibrosis in response to chronic injury mimics the process of wound healing [23] , we asked whether the level of GIV expression is altered during the course of chronic liver injury in patients with chronic HCV hepatitis, a leading cause of liver cirrhosis [24] . We found that full-length GIV mRNA was virtually undetectable in normal livers, but elevated ~50-fold in livers with mild to moderate fibrosis (Ishak score 1–4), and ~175-fold in those with cirrhosis (Ishak scores 5, 6; Fig. 1a ), indicating that GIV mRNA expression increases with increasing degree of liver fibrosis. When we analysed liver samples from two well-accepted animal models for chronic liver injury [25] , that is, surgical bile duct ligation (BDL) and chronic injection of carbon tetrachloride (CCl 4 ), we found that GIV mRNA was virtually undetectable in normal murine livers (sham and vehicle controls) but elevated ~15- to 45-fold in response to both types of injuries during progressive fibrosis ( Fig. 1b,c ). Next we analysed total liver lysates from BDL or CCl 4 -treated mice for GIV protein expression by immunoblotting with an antibody that recognizes the C terminus of full-length GIV (CT-Ab) [26] . GIV was detected exclusively after injury in both study models, increasing with progressive fibrosis ( Fig. 1d,e , Supplementary Fig. 1A ), and such expression correlated with increased activation of the PI3K-Akt pathway, as determined by Akt phosphorylation ( Fig. 1d,e ). GIV was also detected using immunohistochemistry (IHC) in mouse livers exclusively after BDL or CCl 4 injury ( Fig. 1f ), and in liver biopsies from patients with liver fibrosis because of a variety of chronic injuries ( Fig. 1g ). The staining pattern in injured livers was consistent with restricted expression of full-length GIV exclusively in non-parenchymal, that is, interstitial cells, whereas hepatocytes, which comprise ~85% of the total cell mass of the liver, do not express full-length GIV regardless of injury. These findings indicate that (1) there is little or no expression of full-length GIV (neither mRNA nor protein) in normal livers; (2) GIV expression is consistently induced after a variety of chronic injuries; (3) the abundance of GIV mRNA increases with progressive fibrosis; (4) the increase in mRNA is accompanied by translation of GIV protein; and (5) increased GIV protein expression correlates with increased Akt activation in the injured livers. 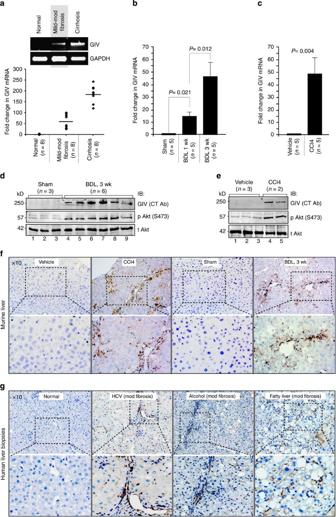Figure 1: Expression of GIV increases in the liver after chronic fibrogenic injury. (a) GIV mRNA levels were analysed in livers from normal and HCV-infected patients with variable degrees of fibrosis using semiquantitative (top) and quantitative PCR (bottom). Representative results for semiquantitative PCR and a scattergram showing the fold induction of GIV mRNA are shown. Horizontal bar=mean.n=number of animals. (b,c) GIV mRNA levels were analysed in livers of mice subjected to BDL or sham surgery (b), or chronic injections of CCl4or vehicle control (c) using qPCR as ina. Results are shown as fold change compared with sham- and vehicle-treated controls. Error bars represent mean±s.d.n=number of animals. Statistical significance was assessed with two-tailed Student’st-test. (d,e) Total liver lysates from mice subjected to BDL or sham surgery (d) chronic injections of CCl4or vehicle control (e) were analysed for full-length GIV, phospho-Akt (pAkt) and total Akt (tAkt) by immunoblotting (IB). (f) FFPE liver sections from mice subjected to BDL or CCl4injury and their respective controls were analysed for expression of full-length GIV protein (CT-Ab) using IHC. Boxed area in top panel is magnified in bottom panels. Magnification= × 10. (g) FFPE liver sections from normal subjects or from patients with a variety of chronic liver injuries were analysed for GIV as ine. Images are representative of 4–11 livers analysed in each category. Boxed area in top panel is magnified in bottom panels. Magnification= × 10. Figure 1: Expression of GIV increases in the liver after chronic fibrogenic injury. ( a ) GIV mRNA levels were analysed in livers from normal and HCV-infected patients with variable degrees of fibrosis using semiquantitative (top) and quantitative PCR (bottom). Representative results for semiquantitative PCR and a scattergram showing the fold induction of GIV mRNA are shown. Horizontal bar=mean. n =number of animals. ( b , c ) GIV mRNA levels were analysed in livers of mice subjected to BDL or sham surgery ( b ), or chronic injections of CCl 4 or vehicle control ( c ) using qPCR as in a . Results are shown as fold change compared with sham- and vehicle-treated controls. Error bars represent mean±s.d. n =number of animals. Statistical significance was assessed with two-tailed Student’s t -test. ( d , e ) Total liver lysates from mice subjected to BDL or sham surgery ( d ) chronic injections of CCl 4 or vehicle control ( e ) were analysed for full-length GIV, phospho-Akt (pAkt) and total Akt (tAkt) by immunoblotting (IB). ( f ) FFPE liver sections from mice subjected to BDL or CCl 4 injury and their respective controls were analysed for expression of full-length GIV protein (CT-Ab) using IHC. Boxed area in top panel is magnified in bottom panels. Magnification= × 10. ( g ) FFPE liver sections from normal subjects or from patients with a variety of chronic liver injuries were analysed for GIV as in e . Images are representative of 4–11 livers analysed in each category. Boxed area in top panel is magnified in bottom panels. Magnification= × 10. Full size image Unlike chronic injuries, when microarrays performed on a variety of acute liver injuries were analysed for the expression profile of GIV, we found that GIV expression was elevated in some, but not all, cases ( Supplementary Fig. 1B–E ). GIV mRNA was minimally upregulated in patients with acute viral hepatitides ( Supplementary Fig. 1B,C ), which carries the potential of progressing to chronicity and liver fibrosis in some patients, whereas no such upregulation was observed in acute alcoholic hepatitis or in a murine model of acute injury by partial hepatectomy ( Supplementary Fig. 1D,E ), two conditions that heal without fibrosis [27] . These findings indicate that GIV expression is induced during some, but not all, injuries of the liver, and that persistent upregulation of GIV expression is primarily restricted only to chronic injuries of the liver. GIV expression is upregulated in activated HSCs To determine which non-parenchymal cell type within the liver contributes to the observed increase in GIV, we carried out liver cell fractionation from BDL-treated and control mice and analysed the isolated cell types for expression of GIV mRNA. Consistent with our IHC staining pattern, we found that hepatocytes have no detectable full-length GIV transcript regardless of injury ( Fig. 2a ). Low levels of GIV mRNA were detected in all the other cells isolated from control livers, which significantly increased after BDL. Both HSCs and Kupffer cells (KCs; the liver-resident macrophages), which drive liver fibrosis in response to chronic liver injury [28] , showed significant increases after injury. We focused on the role of GIV expression in HSCs for two outstanding reasons: (1) they contribute to ~80% collagen produced during liver fibrosis and (2) they are the final common target of cytokines and growth factors produced by other cells that contribute to liver fibrosis, for example, KCs and sinusoidal endothelial cells (ECs) [28] , [29] . When we quantitatively assessed GIV mRNA in isolated HSCs after BDL or CCl 4 injuries, we found, similar to our results in whole liver, that expression of full-length GIV is upregulated approximately two to fourfold during progressive fibrosis in both models of chronic injury ( Fig. 2b,c ). 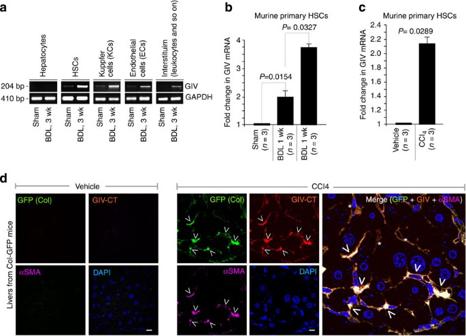Figure 2: Expression of full-length GIV mRNA and protein increases in HSCs after injury. (a) Isolated cell fractions from livers of mice subjected to BDL or sham surgery were analysed for GIV and GAPDH mRNA levels using RT–PCR. (b,c) Primary HSCs isolated from livers of mice subjected to BDL or sham surgery (b) or injections of CCl4or vehicle control (c) were analysed for GIV mRNA using qPCR. Results are shown as fold change compared with sham- and vehicle-treated controls, respectively. Error bars represent mean±s.d.n=number of animals. Statistical significance was assessed with two-tailed Student’st-test. (d) Semithin liver sections from Col-GFP mice chronically treated with injections of CCl4or vehicle control were stained for GIV (red), Collagen (GFP, green), α-SMA (purple) and DAPI/DNA (blue) and analysed using confocal microscopy. Arrowheads=α-SMA pos, Col pos, GIV pos (that is, HSCs); Stars=α-SMA neg, GIV pos, likely to be KCs and Sinusoidal ECs. Scale bar=10 μm. Figure 2: Expression of full-length GIV mRNA and protein increases in HSCs after injury. ( a ) Isolated cell fractions from livers of mice subjected to BDL or sham surgery were analysed for GIV and GAPDH mRNA levels using RT–PCR. ( b , c ) Primary HSCs isolated from livers of mice subjected to BDL or sham surgery ( b ) or injections of CCl 4 or vehicle control ( c ) were analysed for GIV mRNA using qPCR. Results are shown as fold change compared with sham- and vehicle-treated controls, respectively. Error bars represent mean±s.d. n =number of animals. Statistical significance was assessed with two-tailed Student’s t -test. ( d ) Semithin liver sections from Col-GFP mice chronically treated with injections of CCl 4 or vehicle control were stained for GIV (red), Collagen (GFP, green), α-SMA (purple) and DAPI/DNA (blue) and analysed using confocal microscopy. Arrowheads=α-SMA pos, Col pos, GIV pos (that is, HSCs); Stars=α-SMA neg, GIV pos, likely to be KCs and Sinusoidal ECs. Scale bar=10 μm. Full size image To further corroborate whether GIV protein is expressed in HSCs after chronic liver injury, we analysed the expression of full-length GIV in situ in semithin sections of livers harvested from control and CCl 4 -treated Col-green-fluorescent protein (GFP) mice using immunofluorescence. We used Col-GFP transgenic mice that express GFP driven by alpha1 (I) collagen promoter [30] because, in these mice, GFP serves as a surrogate marker for collagen expression in whole-liver extracts and in isolated primary HSCs [30] . As anticipated, GFP (collagen) and α-Smooth muscle actin (α-SMA), a bona fide marker for active HSCs [31] , were detected exclusively after injury. GIV was undetectable in the control liver but was detected in activated HSCs, as determined by colocalization with α-SMA ( Fig. 2d ). Expression of GIV correlated with collagen (GFP) expression in these α-SMA-positive HSCs (arrowheads in Fig. 2d ), indicating that upon injury, expression of GIV protein coincides with HSC activation and collagen synthesis. GIV was also detected at lower levels in α-SMA-negative cells that are likely to be ECs or KCs (stars in Fig. 2d ). Together, these results demonstrate that GIV mRNA is upregulated in HSCs after injury and GIV protein is translated after HSC activation. Expression of GIV precedes collagen during HSC activation Next, we investigated the temporal correlation between GIV expression, HSC activation (as determined by α-SMA expression) and collagen production in HSCs isolated from Col-GFP mice. HSCs were activated on plastic culture dishes and monitored for morphologic changes that are characteristic of transdifferentiation and by the abundance of collagen (GFP) synthesis ( Supplementary Fig. 2 ). On day 1, as expected, inactive HSCs contained lipid droplets laden with retinyl esters and did not express collagen; however, ~50% of those collagen-negative cells already expressed GIV ( Fig. 3a ). Both GIV and collagen expression increased robustly in all HSCs on days 3, 5 and 7. Noteworthy, there were no collagen-positive HSCs that did not also express GIV, indicating that GIV expression invariably preceded expression of collagen. An analysis of mRNA levels confirmed that induction of GIV expression precedes collagen and α-SMA expression ( Fig. 3b–e ) during HSC activation; while GIV expression peaks on day 1 expressions of collagen and α-SMA peak on day 3. These results demonstrate that in HSCs activated ex vivo , upregulation of GIV is likely to be an upstream event that precedes HSC activation and collagen synthesis. 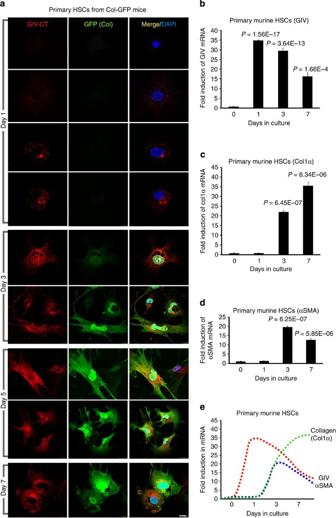Figure 3: Expression of GIV mRNA and protein precedes activation and collagen production in culture-activated HSCs. (a) Primary HSCs isolated from livers of Col-GFP mice were culture-activated on uncoated plastic dishes for 7 days. Cells were fixed at various time points and stained for GIV (red) and DAPI/DNA (blue). Collagen production was detected by GFP signal as a surrogate marker. Representative images on different days are shown. Scale bar=10 μm. (b–e) Primary HSCs isolated from livers of Col-GFP mice were culture-activated on uncoated plastic dishes for 7 days. GIV (b), collagen (c) and α-SMA (d) mRNA levels were measured using qPCR at different time points. (e) Expression patterns of GIV, collagen and α-SMA inb–dare plotted as line graphs superimposed on each other. GIV expression precedes peak expression of α-SMA and collagen. Results are shown as fold change compared with day 0 for each target transcript. Figure 3: Expression of GIV mRNA and protein precedes activation and collagen production in culture-activated HSCs. ( a ) Primary HSCs isolated from livers of Col-GFP mice were culture-activated on uncoated plastic dishes for 7 days. Cells were fixed at various time points and stained for GIV (red) and DAPI/DNA (blue). Collagen production was detected by GFP signal as a surrogate marker. Representative images on different days are shown. Scale bar=10 μm. ( b – e ) Primary HSCs isolated from livers of Col-GFP mice were culture-activated on uncoated plastic dishes for 7 days. GIV ( b ), collagen ( c ) and α-SMA ( d ) mRNA levels were measured using qPCR at different time points. ( e ) Expression patterns of GIV, collagen and α-SMA in b – d are plotted as line graphs superimposed on each other. GIV expression precedes peak expression of α-SMA and collagen. Results are shown as fold change compared with day 0 for each target transcript. Full size image GIV is required for activation of HSCs HSC activation is characterized by the key phenotypes such as enhanced proliferation, cell migration, actin remodelling, resistance to apoptosis and collagen production [1] . Next, we asked whether GIV is required for some or most of these phenotypes and, thereby, for HSC activation. First, we analysed GIV expression, localization and properties in cultured human Lx2 HSC line, which has been extensively characterized and widely accepted as a model system to study fibrogenic pathways [31] . We found that Lx2 cells express GIV as an ~250-kDa full-length protein ( Fig. 4a ) that localizes to the Golgi and plasma membrane (PM)-associated actin bed ( Supplementary Fig. 3A ), as previously shown in other cell lines [19] , [32] . Similar localization was also observed in primary murine HSCs ( Supplementary Fig. 3A ). Compared with control cells, GIV-depleted cells (~85–90% efficacy; Fig. 4a ) showed fewer actin stress fibres ( Fig. 4b ), impaired cell migration ( Fig. 4c , Supplementary Fig. 3B ) and suppressed mitosis, as determined by nuclear accumulation of phospho-histone H3 ( Fig. 4d , Supplementary Fig. 3C ) and by BrDU uptake ( Fig. 4e , Supplementary Fig. 3D ). These results demonstrate that GIV is required for cell migration, proliferation and cytoskeletal remodelling in HSCs. 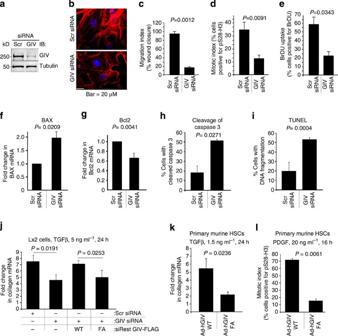Figure 4: GIV is required for actin remodelling, proliferation, migration, survival and collagen production in HSCs. (a) Lx2 cells were treated either with control (Scr) or with G cvcIV siRNA, lysates were analysed for GIV depletion with IB. (b) Control (Scr) and GIV siRNA-treated Lx2 cells were fixed and stained for Phalloidin (red) and DAPI/DNA (blue) and visualized using confocal microscopy. Scale bar=20 μm. (c) Control (Scr) or GIV siRNA-treated Lx2 cells were analysed for their ability to migrate and close a scratch wound by serial imaging of the wound area (seeSupplementary Fig. 3B). Results are expressed as % wound closure. (d,e) Lx2 cells as incwere analysed for nuclear phospho-Histone H3 or BrDU uptake using immunofluorescence and analysed with confocal microscopy (seeSupplementary Fig. 3C,D). Results are expressed as % cells positive for staining. (f,g) Control (Scr) or GIV siRNA-treated Lx2 cells were analysed for BAX (f) and Bcl-2 (g) mRNA using qPCR. Results are displayed as fold change compared with their respective Scr-treated controls. (h,i) Control (Scr) or GIV siRNA-treated Lx2 cells were analysed for cleaved Caspase 3 (i) with immunofluorescence and fragmented DNA with TUNEL staining (h). Bar graphs display % cells with cleaved Caspase 3 (i) or fragmented DNA (h; TUNEL) onyaxis. (j) Lx2 cells were treated with control (Scr) or GIV siRNA or transfected with siRNA-resistant GIV-WT or GIV-FA, as indicated, starved and subsequently treated with TGF-β1. Collagen α1 mRNA was determined using qPCR and results are displayed as fold change compared with starved controls (yaxis). (k,l) Primary murine HSCs were infected with adenoviruses expressing HA-tagged GIV-WT or GIV-FA, starved and subsequently treated with TGF-β1 (i) or PDGF-BB (j). Collagen α1 mRNA level was determined using qPCR. Results are displayed as fold change compared with starved controls (yaxis) (i) and mitotic index was analysed using phospho-Histone H3 (j) as ind. Results are displayed as % of cells positive for nuclear phospho-Histone H3 (yaxis). Error bars represent mean±s.d.n=3. Statistical significance was assessed with two-tailed Student’st-test. Figure 4: GIV is required for actin remodelling, proliferation, migration, survival and collagen production in HSCs. ( a ) Lx2 cells were treated either with control (Scr) or with G cvcIV siRNA, lysates were analysed for GIV depletion with IB. ( b ) Control (Scr) and GIV siRNA-treated Lx2 cells were fixed and stained for Phalloidin (red) and DAPI/DNA (blue) and visualized using confocal microscopy. Scale bar=20 μm. ( c ) Control (Scr) or GIV siRNA-treated Lx2 cells were analysed for their ability to migrate and close a scratch wound by serial imaging of the wound area (see Supplementary Fig. 3B ). Results are expressed as % wound closure. ( d , e ) Lx2 cells as in c were analysed for nuclear phospho-Histone H3 or BrDU uptake using immunofluorescence and analysed with confocal microscopy (see Supplementary Fig. 3C,D ). Results are expressed as % cells positive for staining. ( f , g ) Control (Scr) or GIV siRNA-treated Lx2 cells were analysed for BAX ( f ) and Bcl-2 ( g ) mRNA using qPCR. Results are displayed as fold change compared with their respective Scr-treated controls. ( h , i ) Control (Scr) or GIV siRNA-treated Lx2 cells were analysed for cleaved Caspase 3 ( i ) with immunofluorescence and fragmented DNA with TUNEL staining ( h ). Bar graphs display % cells with cleaved Caspase 3 ( i ) or fragmented DNA ( h ; TUNEL) on y axis. ( j ) Lx2 cells were treated with control (Scr) or GIV siRNA or transfected with siRNA-resistant GIV-WT or GIV-FA, as indicated, starved and subsequently treated with TGF-β1. Collagen α1 mRNA was determined using qPCR and results are displayed as fold change compared with starved controls ( y axis). ( k , l ) Primary murine HSCs were infected with adenoviruses expressing HA-tagged GIV-WT or GIV-FA, starved and subsequently treated with TGF-β1 ( i ) or PDGF-BB ( j ). Collagen α1 mRNA level was determined using qPCR. Results are displayed as fold change compared with starved controls ( y axis) ( i ) and mitotic index was analysed using phospho-Histone H3 ( j ) as in d . Results are displayed as % of cells positive for nuclear phospho-Histone H3 ( y axis). Error bars represent mean±s.d. n =3. Statistical significance was assessed with two-tailed Student’s t -test. Full size image As activated HSCs acquire resistance to apoptosis [1] , we analysed the expression of two bona fide pro- (Bax) and anti (Bcl-2)-apoptotic signalling intermediates [33] . In GIV-depleted HSCs, pro-apoptotic Bax was upregulated approximately twofold ( Fig. 4f ) and anti-apoptotic Bcl-2 was decreased by ~40% ( Fig. 4g ) compared with controls, indicating that in the absence of GIV cells are overall pro-apoptotic. Moreover, in HSCs treated with gliotoxin [34] , an inducer of apoptosis, GIV expression was reduced by ~50%, alongside the expected increase in Bax and decrease in Bcl-2 ( Supplementary Fig. 3E ), indicating that changes in GIV expression profile after a pro-apoptotic injury mirrors that of an anti-apoptotic gene, that is, Bcl-2, and not Bax. To confirm GIV’s anti-apoptotic role in HSCs, we carried out TdT-mediated dUTP nick end labelling (TUNEL) assays and analysed cleavage of Caspase 3, two widely used approaches for measuring cellular apoptosis [35] . We found that compared with control cells, GIV-depleted cells had increased Caspase 3 activity, as determined by the presence of the cleaved enzyme ( Fig. 4h ; ~2.5-fold) and increased, fragmented DNA, as determined using TUNEL ( Fig. 4i ; ~2.5-fold). These results demonstrate that depletion of GIV triggers apoptosis, and that GIV is required for survival of HSCs after injury. As GIV modulates signal transduction primarily via its GEF property [16] , we asked whether two key HSC phenotypes, that is, proliferation and collagen production, require GIV’s GEF function. To investigate this, we took advantage of previously validated GIV constructs: wild-type GIV (GIV-WT) and GEF-deficient F1685A (GIV-FA) mutant [16] . Depletion of GIV from Lx2 HSCs suppressed collagen production in response to TGF-β1 by ~40–50% compared with controls ( Fig. 4j ), an effect that was reversed by exogenous expression of short interfering (siRNA)-resistant GIV-WT, but not by GIV-FA mutant. Similar results were obtained also in TGF-β1-stimulated primary HSCs, that is, expression of GIV-FA suppressed collagen synthesis by ~60% compared with GIV-WT ( Fig. 4k ). Finally, with regard to mitogenic response to PDGF, expression of GIV-FA suppressed mitosis by approximately sevenfold compared with GIV-WT ( Fig. 4l ), indicating that GIV’s GEF function is required for growth factor-stimulated collagen synthesis and proliferation in HSCs. Together, these results demonstrate that GIV and its GEF function are required for several key phenotypes that are critical for transdifferentiation and sustained activation of HSCs during progressive fibrosis. PDGFRβ binds and phosphorylates GIV in activated HSCs Next, we asked which receptor(s) and ligands activate GIV-dependent signalling to potentiate HSC activation. First, we analysed signalling events triggered in Lx2 cells by PDGF and TGF-β1, the two major profibrotic stimuli [2] , [3] . We found that PDGF, but not TGFβ-1, triggered phosphorylation of GIV at Tyr(Y)1764, a substrate site for RTKs [17] and Ser(S)1416, a substrate site for Akt [32] , that are established surrogate markers of activation of the RTK-GIV-PI3K-Akt signalling pathway [17] ( Fig. 5a,b ). However, both growth factors triggered phosphorylation of Akt, SMAD and ERK proteins ( Fig. 5a,b ). Consistent with such activation, GIV co-immunoprecipitated with ligand-activated PDGFRβ ( Fig. 5c ), along with Gαi and PI3K. Using recombinant proteins in pull-down assays we confirmed that the interaction between autophosphorylated PDGFRβ and GIV’s C terminus is direct ( Fig. 5d ) and found that recombinant PDGFRβ phosphorylated GIV on tyrosines 1.764 and 1,798 in vitro ( Fig. 5e ), the same residues that are targeted by other RTKs [17] . We found that tyrosine-phosphorylated GIV partially colocalized with activated PDGFRβ on patches at the PM in culture-activated primary HSCs (arrowheads, Fig. 5f ), as well as in PDGF-stimulated Lx2 cells (arrowheads, Fig. 5g ). These results demonstrate that upon PDGF stimulation, GIV and Gαi interact with activated PDGFRβ, presumably at the PM. Subsequent phosphorylation of GIV by PDGFR triggers the previously defined RTK(active)-pTyrGIV-Gi-PI3K pathway [17] . By contrast, neither GIV nor Gαi could be detected in complex with TGFβR under the same conditions, suggesting that the Ser/Thr TGFβR kinase may not bind or directly transduce signal via GIV. 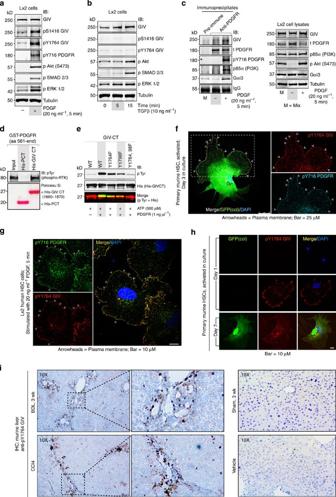Figure 5: PDGFRβ directly binds and phosphorylates GIV in HSCs during liver injury. (a,b) Whole-cell lysates of Lx2 cells stimulated with either PDGF-BB (a) or with TGF-β1 (b) were analysed for various signalling pathways using IB. (c) Immunoprecipitation was carried out on lysates (right panel) of serum-starved or PDGF-BB-treated Lx2 cells with anti-PDGFR or control IgG. Bound immune complexes (left) were analysed for GIV, total (t) and activated (pY716) PDGFR, p85α(PI3K) and Gαi3 by IB. M=Mix of starved and stimulated Lx2 lysates. (d) GST-PDGFR was autophosphorylatedin vitroand used in pull-down assays with purified His-GIV-CT or His-PCT (Podocalyxin Tail; a negative control). Bound receptor was visualized by IB using phospho-Tyr (pTyr) antibody. Equal amounts of His-tagged ligands were confirmed with Ponceau S stain. (e)In vitrokinase assays were carried out with recombinant PDGFR on WT and phospho-mutants of His-GIV-CT. Reactions were analysed for pTyr and His-GIV-CT by IB. Yellow pixels in the merged panel (pTyr and His) shows phosphoGIV-CT. (f) Culture-activated primary HSCs from Col-GFP mice were fixed and stained for active pY1764GIV (red) and active pY716PDGFR (cyan). Merge panel shows colocalization of red and cyan pixels at the PM (arrowheads). Arrowheads=PM. Scale bar=25 μm. (g) Lx2 cells stimulated with PDGF-BB were fixed and stained for pY1764GIV (red), active pY716PDGFR (green) and DAPI/DNA (blue). Merge panel shows yellow pixels indicative of colocalization at the PM (arrowheads). Arrowheads=Plasma membrane. Scale bar=10 μm. (h) Culture-activated primary HSCs were fixed and stained for active pY1764GIV (red) and DAPI/DNA (blue). Collagen production was detected with GFP signal. Scale bar=10 μm.f–hwere analysed with confocal microscopy. (i) Left: liver sections from mice subjected to BDL or CCl4injury were analysed for active pY1764GIV using IHC. Boxed area on left panels are magnified on the right. Right: no staining was observed in the respective controls for both experimental models. Magnification= × 10. Figure 5: PDGFRβ directly binds and phosphorylates GIV in HSCs during liver injury. ( a , b ) Whole-cell lysates of Lx2 cells stimulated with either PDGF-BB ( a ) or with TGF-β1 ( b ) were analysed for various signalling pathways using IB. ( c ) Immunoprecipitation was carried out on lysates (right panel) of serum-starved or PDGF-BB-treated Lx2 cells with anti-PDGFR or control IgG. Bound immune complexes (left) were analysed for GIV, total (t) and activated (pY716) PDGFR, p85α(PI3K) and Gαi3 by IB. M=Mix of starved and stimulated Lx2 lysates. ( d ) GST-PDGFR was autophosphorylated in vitro and used in pull-down assays with purified His-GIV-CT or His-PCT (Podocalyxin Tail; a negative control). Bound receptor was visualized by IB using phospho-Tyr (pTyr) antibody. Equal amounts of His-tagged ligands were confirmed with Ponceau S stain. ( e ) In vitro kinase assays were carried out with recombinant PDGFR on WT and phospho-mutants of His-GIV-CT. Reactions were analysed for pTyr and His-GIV-CT by IB. Yellow pixels in the merged panel (pTyr and His) shows phosphoGIV-CT. ( f ) Culture-activated primary HSCs from Col-GFP mice were fixed and stained for active pY1764GIV (red) and active pY716PDGFR (cyan). Merge panel shows colocalization of red and cyan pixels at the PM (arrowheads). Arrowheads=PM. Scale bar=25 μm. ( g ) Lx2 cells stimulated with PDGF-BB were fixed and stained for pY1764GIV (red), active pY716PDGFR (green) and DAPI/DNA (blue). Merge panel shows yellow pixels indicative of colocalization at the PM (arrowheads). Arrowheads=Plasma membrane. Scale bar=10 μm. ( h ) Culture-activated primary HSCs were fixed and stained for active pY1764GIV (red) and DAPI/DNA (blue). Collagen production was detected with GFP signal. Scale bar=10 μm. f – h were analysed with confocal microscopy. ( i ) Left: liver sections from mice subjected to BDL or CCl 4 injury were analysed for active pY1764GIV using IHC. Boxed area on left panels are magnified on the right. Right: no staining was observed in the respective controls for both experimental models. Magnification= × 10. Full size image Next we investigated the temporal correlation between activation of the RTK(active)-pTyrGIV-PI3K pathway (using phosphoTyr 1764 GIV as a surrogate marker) and collagen synthesis in culture-activated primary HSCs. On day 1, when collagen is still undetectable, pY1764GIV is detected in ~50% of HSCs ( Fig. 5h , Supplementary Fig. 4 ). By day 3, ~15–20% HSCs express collagen, whereas 100% express pY1764GIV ( Supplementary Fig. 4 ). Thus, early expression of GIV during HSC activation that we observed before ( Fig. 3a ) is also accompanied by activation of the PDGFR-GIV-PI3K pathway, and both are upstream events that precede collagen synthesis during HSC activation. We confirmed that this pathway is activated in vivo during liver fibrosis because pY1764GIV was detected exclusively in livers from BDL or CCl 4 -treated mice and not in control livers using IHC ( Fig. 5i ). These results demonstrate that upon ligand stimulation, GIV directly binds autophosphorylated PDGFRβ, which allows: (a) GIV to link G protein activation to RTK signalling, and (b) phosphorylation of GIV by PDGFRβ, two events that synergistically enhance Akt signals via GIV [17] . GIV enhances profibrotic signals downstream of multiple receptors As the PI3K-Akt and TGFβ-SMAD pathways are major profibrotic signals that drive liver fibrosis [36] , we asked whether GIV and, more specifically, its GEF function or tyrosine phosphorylation modulate these signals in HSCs. To investigate this, we took advantage of two more previously validated GIV constructs: non-phosphorylatable Y1764/1798F mutant (GIV-YF) and GIV-FA/YF in which both GEF and tyrosines are mutated. We found that exogenous expression of GIV-WT, but not the mutants in Lx2 cells, enhanced phosphorylation of both Akt and SMAD 2/3 proteins ( Fig. 6a ), indicating that both GIV’s GEF function and tyrosine phosphorylation are essential. Depletion of endogenous GIV in Lx2 cells suppressed Akt phosphorylation ( Fig. 6b ), an effect reversed by exogenous expression of siRNA-resistant GIV-WT, but not GIV-FA ( Fig. 6b ), indicating that GIV’s GEF function is required for maximal enhancement of Akt phosphorylation in HSCs. GIV’s GEF function was also required for enhancement of Akt phosphorylation in response to a variety of ligands (serum, PDGF-BB, TGF-β1, RANTES, which activates CCRs, and lipopolysaccharide (LPS). which activates Toll-like receptors, TLR4) that target fibrogenic receptors of diverse classes ( Fig. 6c,d ), indicating that GIV enhances the profibrotic PI3K-Akt pathway downstream of multiple receptors via its GEF function. FoxO1, a major downstream target of Akt, whose inactivation and nuclear exclusion triggers HSC transdifferentiation during liver fibrosis [10] , was excluded from the nucleus in ~92% of the cells expressing GIV-WT ( Fig. 6e,f ). By contrast, in cells expressing GIV-FA, FoxO1 was seen in the nucleus in ~50% of the cells, indicating that GIV’s GEF function is required for nuclear exclusion and inactivation of FoxO1. Furthermore, compared with cells expressing GIV-WT, those expressing GIV-FA displayed fewer stress fibres ( Supplementary Fig. 5 ), an overall pro-apoptotic phenotype [lower Bcl-2 ( Fig. 6g ) and higher BAX ( Fig. 6h ), higher Caspase 3 activity ( Fig. 6i ) and more abundance of fragmented DNA analysed using TUNEL ( Fig. 6j )], lower SMAD 2/3 activation, based on its decreased phosphorylation ( Fig. 6k ) and reduced nuclear localization ( Fig. 6l,m ). Taken together, these results demonstrate that GIV’s GEF function is essential for the key profibrogenic phenotypes that characterize HSC activation: actin cytoskeletal remodelling, HSC survival and enhanced PI3K-Akt-FoxO1 and the TGFβ-SMAD pathways. 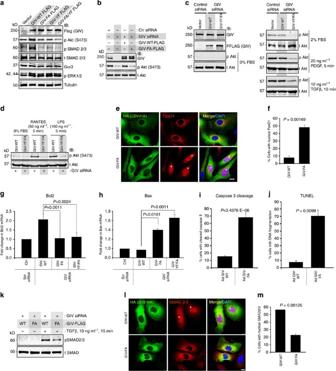Figure 6: GIV’s GEF function enhances profibrogenic Akt and SMAD signals in HSCs. (a) Whole-cell lysates of Lx2 cells expressing GIV mutants were analysed for various signalling pathways by IB. (b–d) Lx2 cells treated with control (Scr) or GIV siRNA were transfected with siRNA-resistant GIV-WT or the indicated mutants, starved (0% FBS), and then stimulated with serum or various ligands before lysis. Equal aliquots of lysates were analysed for GIV, phospho- and total Akt by IB. (e,f) Lx2 cells infected with GIV-WT-HA or GIV-FA-HA adenoviruses were maintained in 0.2% FBS, fixed and stained for HA (GIV, green), FoxO1 (red) and DAPI/DNA (blue) and analysed using confocal microscopy. Star=nuclear FoxO1. Scale bar=10 μm. Results display % cells with nuclear FoxO1 (yaxis) (f). (g,h) Lx2 cells depleted of endogenous GIV were subsequently transfected with various GIV constructs, and RNA extracted of these cells were analysed for Bcl-2 (g) and BAX (h) mRNA levels using qPCR. (i,j) Lx2 cells were infected with GIV-WT-HA or GIV-FA-HA adenoviruses, maintained in 0 % FBS, fixed and analysed for cleaved Caspase 3 (j) with immunofluorescence and for fragmented DNA with TUNEL staining (i). Bar graphs display % cells with cleaved Caspase 3 (j) or fragmented DNA (i; TUNEL) onyaxis. (k) Lx2 cells depleted of endogenous GIV were subsequently transfected with siRNA-resistant GIV-WT or GIV-FA, stimulated with TGFβ and phospho- (p)SMAD and total (t)SMAD 2/3 were analysed by IB. The ratio of pSMAD/tSMAD was approximately twofold higher in cells expressing GIV-WT than in those expressing GIV-FA, as determined using band densitometry. (l,m) Lx2 cells infected with GIV-WT-HA or GIV-FA-HA adenoviruses were maintained in 0.2% FBS, fixed and stained for HA (GIV, green), SMAD 2/3 (red) and DAPI/DNA (blue) and analysed using confocal microscopy. Star=nuclear SMAD 2/3. Scale bar=10 μm. (m) Bar graphs display % cells with nuclear tSMAD2/3 ink. Error bars represent mean±s.d.n=3. Statistical significance was assessed with two-tailed Student’st-test. Figure 6: GIV’s GEF function enhances profibrogenic Akt and SMAD signals in HSCs. ( a ) Whole-cell lysates of Lx2 cells expressing GIV mutants were analysed for various signalling pathways by IB. ( b – d ) Lx2 cells treated with control (Scr) or GIV siRNA were transfected with siRNA-resistant GIV-WT or the indicated mutants, starved (0% FBS), and then stimulated with serum or various ligands before lysis. Equal aliquots of lysates were analysed for GIV, phospho- and total Akt by IB. ( e , f ) Lx2 cells infected with GIV-WT-HA or GIV-FA-HA adenoviruses were maintained in 0.2% FBS, fixed and stained for HA (GIV, green), FoxO1 (red) and DAPI/DNA (blue) and analysed using confocal microscopy. Star=nuclear FoxO1. Scale bar=10 μm. Results display % cells with nuclear FoxO1 ( y axis) ( f ). ( g , h ) Lx2 cells depleted of endogenous GIV were subsequently transfected with various GIV constructs, and RNA extracted of these cells were analysed for Bcl-2 ( g ) and BAX ( h ) mRNA levels using qPCR. ( i , j ) Lx2 cells were infected with GIV-WT-HA or GIV-FA-HA adenoviruses, maintained in 0 % FBS, fixed and analysed for cleaved Caspase 3 ( j ) with immunofluorescence and for fragmented DNA with TUNEL staining ( i ). Bar graphs display % cells with cleaved Caspase 3 ( j ) or fragmented DNA ( i ; TUNEL) on y axis. ( k ) Lx2 cells depleted of endogenous GIV were subsequently transfected with siRNA-resistant GIV-WT or GIV-FA, stimulated with TGFβ and phospho- (p)SMAD and total (t)SMAD 2/3 were analysed by IB. The ratio of pSMAD/tSMAD was approximately twofold higher in cells expressing GIV-WT than in those expressing GIV-FA, as determined using band densitometry. ( l , m ) Lx2 cells infected with GIV-WT-HA or GIV-FA-HA adenoviruses were maintained in 0.2% FBS, fixed and stained for HA (GIV, green), SMAD 2/3 (red) and DAPI/DNA (blue) and analysed using confocal microscopy. Star=nuclear SMAD 2/3. Scale bar=10 μm. ( m ) Bar graphs display % cells with nuclear tSMAD2/3 in k . Error bars represent mean±s.d. n =3. Statistical significance was assessed with two-tailed Student’s t -test. Full size image GIV inhibits antifibrotic signals downstream of multiple receptors Next, we asked whether activation of Gαi via GIV’s GEF function modulates antifibrotic cAMP signals during HSC activation. First, we confirmed that GIV expressed in HSCs bound G proteins as expected for a GEF [16] , [19] , that is, it preferentially bound inactive Gαi3 (GDP loaded; Fig. 7a ), and not to Gαi3 in active conformation (loaded with GDP + AlF 4 − ) in GST pulldown assays. Next, we confirmed that various stimuli that require GIV’s GEF function to enhance Akt ( Fig. 6d,e ) can also trigger the activation of Gαi3 in Lx2 cells ( Fig. 7b ), as determined by an antibody that specifically recognizes the active GTP-bound conformation of Gαi [37] . Depletion of endogenous GIV suppressed Gαi3 activity ( Fig. 7c ), an effect reversed by exogenous expression of siRNA-resistant GIV-WT, but not GIV-FA, indicating that GIV’s GEF function is required for activation of Gαi3 in HSCs. As expected, loss of Gαi3 activity in HSCs expressing GIV-FA was accompanied by increased accumulation of cellular cAMP ( Fig. 7d ) and enhanced phosphorylation ( Fig. 7e ) and nuclear translocation ( Fig. 7f,g ) of its downstream target, CREB, indicating that GIV’s GEF function is required for inhibition of the cAMP-CREB pathway. These results demonstrate that GIV inhibits the antifibrogenic cAMP pathway in HSCs via its GEF function. 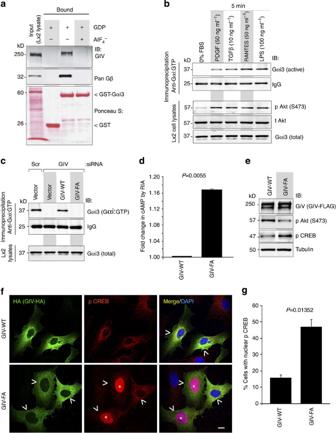Figure 7: GIV activates Gαi and suppresses the antifibrogenic cAMP/PKA/pCREB signals in HSCs. (a) Lysates of Lx2 cells were used as the source of full-length GIV in pull-down assays with GST or GST-Gαi3 preloaded with GDP alone (inactive) or with AlF4−(active) and immobilized on glutathione beads. Bound GIV and Gβγ were analysed by IB. The GST proteins are shown with Ponceau S stain. (b) Serum-starved Lx2 cells were stimulated with a variety of ligands before lysis. Equal aliquots of lysates were subjected to immunoprecipitation with Gαi:GTP mAb, which recognizes active conformation of the G protein and immune complexes were analysed for Gαi3 by IB. (c) Lx2 cells treated with control (Scr) or GIV siRNA were transfected with siRNA-resistant GIV-WT or GIV-FA and maintained in 0.2% FBS. Lysates were analysed for active Gαi3 as inb. (d) Lx2 cells transfected with GIV-WT or GIV-FA were stimulated with PDGF-BB before lysis. Lysates were analysed for cAMP using radioimmunoassay and normalized to total protein. Results are displayed as fold change in cAMP (yaxis). (e) Lx2 cells transfected with GIV-WT or GIV-FA were analysed for GIV, phospho(p)Akt, phospho(p)CREB and tubulin by IB. The ratio of pCREB/tubulin was ~2.5-fold higher in cells expressing GIV-FA than in those expressing GIV-WT, as determined using band densitometry. (f) Lx2 cells infected with GIV-WT-HA or GIV-FA-HA adenoviruses were maintained in 0.2% FBS, fixed and stained for hemagglutinin (HA) (GIV, green), phospho(p)CREB (red) and DAPI/DNA (blue) and analysed using confocal microscopy. Arrowhead=GIV-expressing cell. Star=nuclear p CREB. Scale bar=10 μm. Results display % cells with nuclear pCREB (yaxis) (g). Error bars represent mean±s.d.n=3. Statistical significance was assessed with two-tailed Student’st-test. Figure 7: GIV activates Gαi and suppresses the antifibrogenic cAMP/PKA/pCREB signals in HSCs. ( a ) Lysates of Lx2 cells were used as the source of full-length GIV in pull-down assays with GST or GST-Gαi3 preloaded with GDP alone (inactive) or with AlF 4 − (active) and immobilized on glutathione beads. Bound GIV and Gβγ were analysed by IB. The GST proteins are shown with Ponceau S stain. ( b ) Serum-starved Lx2 cells were stimulated with a variety of ligands before lysis. Equal aliquots of lysates were subjected to immunoprecipitation with Gαi:GTP mAb, which recognizes active conformation of the G protein and immune complexes were analysed for Gαi3 by IB. ( c ) Lx2 cells treated with control (Scr) or GIV siRNA were transfected with siRNA-resistant GIV-WT or GIV-FA and maintained in 0.2% FBS. Lysates were analysed for active Gαi3 as in b . ( d ) Lx2 cells transfected with GIV-WT or GIV-FA were stimulated with PDGF-BB before lysis. Lysates were analysed for cAMP using radioimmunoassay and normalized to total protein. Results are displayed as fold change in cAMP ( y axis). ( e ) Lx2 cells transfected with GIV-WT or GIV-FA were analysed for GIV, phospho(p)Akt, phospho(p)CREB and tubulin by IB. The ratio of pCREB/tubulin was ~2.5-fold higher in cells expressing GIV-FA than in those expressing GIV-WT, as determined using band densitometry. ( f ) Lx2 cells infected with GIV-WT-HA or GIV-FA-HA adenoviruses were maintained in 0.2% FBS, fixed and stained for hemagglutinin (HA) (GIV, green), phospho(p)CREB (red) and DAPI/DNA (blue) and analysed using confocal microscopy. Arrowhead=GIV-expressing cell. Star=nuclear p CREB. Scale bar=10 μm. Results display % cells with nuclear pCREB ( y axis) ( g ). Error bars represent mean±s.d. n =3. Statistical significance was assessed with two-tailed Student’s t -test. Full size image Taken together, we propose ( Fig. 8 ) that GIV serves as a central hub that integrates signals downstream of multiple fibrogenic receptors and simultaneously enhances the profibrotic (PI3K-Akt-FoxO1 and TGFβ-SMAD) and inhibits the antifibrotic (cAMP-PKA-pCREB) pathways to shift the delicate balance between pro- and antifibrogenic signalling to an overall profibrotic signalling programme that favours fibrosis. Consequently, phenotypes that are critical for sustained activation of HSCs and collagen synthesis are enhanced through a combination of transcriptional (via FoxO1, SMAD and CREB) and non-transcriptional mechanisms (via PI3K, Akt and cytoskeletal remodelling). 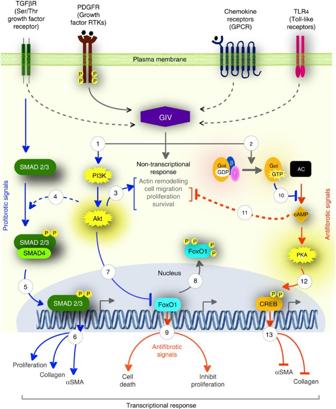Figure 8: GIV enhances profibrogenic and inhibits antifibrogenic signalling pathways in HSCs. Ligand stimulation of diverse classes of fibrogenic receptors (top) converges upon GIV either via direct interaction (solid arrow) or via unknown mechanism (interrupted arrow) to enhance PI3K-Akt signalling (1) and activate trimeric Gαi (2). GIV-dependent activation of Akt elicits several non-transcriptional responses (3) that lead to activation of HSCs. The GIV-PI3K-Akt pathway also modulates two distinct transcriptional programmes—(i) potentiation of the profibrotic TGFβ-SMAD pathway by increasing phosphorylation of SMAD 2/3 (4) and its translocation into the nucleus (5), and thereby enhancing proliferation and transcription of collagen and α-SMA (6); (ii) inhibition of the transcription factor FoxO1 by phosphorylation (7) and by triggering its translocation outside the nucleus (8), thereby antagonizing the antifibrotic programme (9) that FoxO1 maintains in physiology. Activation of Gi by GIV’s GEF function (2) inhibits the production of cAMP (10), a major antifibrotic pathway in HSCs by virtue of its ability to inhibit HSC migration and proliferation (11). The cAMP-PKA pathway is also known to inhibit fibrosis at a transcriptional level by phosphorylating CREB (12) that translocates to the nucleus and inhibits transcription of collagen and α-SMA (13). Profibrogenic pathways=blue; antifibrogenic=red. Figure 8: GIV enhances profibrogenic and inhibits antifibrogenic signalling pathways in HSCs. Ligand stimulation of diverse classes of fibrogenic receptors (top) converges upon GIV either via direct interaction (solid arrow) or via unknown mechanism (interrupted arrow) to enhance PI3K-Akt signalling (1) and activate trimeric Gαi (2). GIV-dependent activation of Akt elicits several non-transcriptional responses (3) that lead to activation of HSCs. The GIV-PI3K-Akt pathway also modulates two distinct transcriptional programmes—(i) potentiation of the profibrotic TGFβ-SMAD pathway by increasing phosphorylation of SMAD 2/3 (4) and its translocation into the nucleus (5), and thereby enhancing proliferation and transcription of collagen and α-SMA (6); (ii) inhibition of the transcription factor FoxO1 by phosphorylation (7) and by triggering its translocation outside the nucleus (8), thereby antagonizing the antifibrotic programme (9) that FoxO1 maintains in physiology. Activation of Gi by GIV’s GEF function (2) inhibits the production of cAMP (10), a major antifibrotic pathway in HSCs by virtue of its ability to inhibit HSC migration and proliferation (11). The cAMP-PKA pathway is also known to inhibit fibrosis at a transcriptional level by phosphorylating CREB (12) that translocates to the nucleus and inhibits transcription of collagen and α-SMA (13). Profibrogenic pathways=blue; antifibrogenic=red. Full size image Elevated GIV expression indicates progression of fibrosis As GIV is upregulated early during liver fibrosis and its expression is required for HSC activation, we hypothesized that detection of GIV in liver biopsies could indicate sustained activation of HSCs and mark the potential for progression to cirrhosis. We tested this hypothesis in liver biopsies obtained from 21 males with chronic HCV infection because the rate of fibrogenic progression in these patients varies markedly, and the need for a biomarker that differentiates rapid from slow progressors still remains unmet [38] . Fibrosis was staged with the Ishak scale (ranging from 0=no fibrosis to 6=cirrhosis) [38] . As shown previously, GIV was undetectable in normal livers ( Fig. 9A,Ba , ) and detected in 100% of livers with moderate to severe fibrosis (scores 3–6) ( Fig. 9A and Bb , ). However, GIV was detected only in ~37% of livers with minimal or no fibrosis (scores=0–2; Fig. 9A,B-c, d , ). Noteworthy, GIV expression did not show any correlation with age, alcohol intake, degrees of inflammation or fatty infiltration. These results demonstrate that some, but not all, patients express GIV during the early stages of chronic viral hepatitis, even before significant fibrosis has occurred, but with the progression to cirrhosis, all are positive. Of the eight patients with minimal or no fibrosis, three patients whose liver biopsies were positive for GIV progressed to advanced fibrosis, as determined with increasing FIB-4 ( Fig. 9C ) and APRI ( Fig. 9D ) scores [39] , [40] during a 3-year follow-up. These results suggest that GIV expression in liver biopsies may predict the progression of fibrosis and thereby serve as a biomarker for the disease. We propose that detection of GIV in liver biopsies early during HCV infection might distinguish those who progress rapidly to cirrhosis from those who progress slowly or not at all. 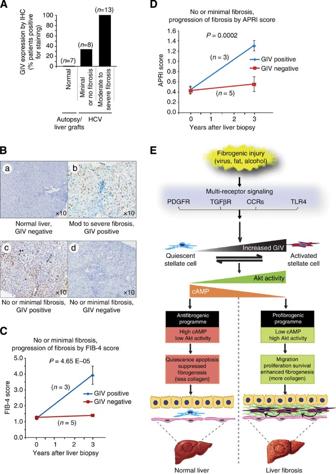Figure 9: GIV expression in liver biopsies may predict fibrogenic progression. (A) GIV expression was analysed in liver biopsies from normal subjects and a cohort of HCV-infected patients at various stages of fibrosis using IHC. Staining was scored by two pathologists blinded to the degree of fibrosis using a simple binary scoring system, that is, positive or negative for GIV. Results are displayed as % patients positive for GIV (yaxis) in each category of fibrosis. (B) Representative IHC images fromAare displayed showing examples of positively and negatively stained liver samples within different categories of fibrosis. Magnification= × 10. (C,D) Line plots depict the progression of fibrosis in patients with no or minimal fibrosis, as determined using FIB-4 (C) and APRI (D) scores derived from clinical parameters at the time of liver biopsy and at 3-year follow-up.Pvalues indicate significant differences in fibrosis scores at 3 years. (E) Schematic shows our proposed model for GIV’s role in fibrogenic signalling in HSCs during liver fibrosis. Top to bottom: fibrogenic injuries of various kinds result in the activation of diverse classes of receptors that trigger upregulation of GIV in HSCs. Increased GIV triggers transformation of quiescent HSCs into activated myofibroblasts by modulating two key signalling pathways: (1) the profibrotic PI3K-Akt pathway and (2) the antifibrotic cAMP-PKA pathway. In quiescent HSCs low levels of GIV expression generate a net antifibrogenic signalling programme characterized by low Akt activity and impaired activation of Gαi with resultant high levels of cAMP. In activated HSCs, high levels of GIV expression generate a net profibrogenic signalling programme characterized by high Akt activity and increased activation of Gαi with resultant low levels of cAMP. Low GIV expression maintains HSCs in quiescent state, triggers apoptosis and suppresses collagen production in the normal liver, whereas high GIV expression enhances HSC migration, proliferation and survival, and triggers collagen production, thereby leading to liver fibrosis.n=number of patients. Error bars represent mean±s.d. Statistical significance was assessed with two-tailed Student’st-test. Figure 9: GIV expression in liver biopsies may predict fibrogenic progression. ( A ) GIV expression was analysed in liver biopsies from normal subjects and a cohort of HCV-infected patients at various stages of fibrosis using IHC. Staining was scored by two pathologists blinded to the degree of fibrosis using a simple binary scoring system, that is, positive or negative for GIV. Results are displayed as % patients positive for GIV ( y axis) in each category of fibrosis. ( B ) Representative IHC images from A are displayed showing examples of positively and negatively stained liver samples within different categories of fibrosis. Magnification= × 10. ( C , D ) Line plots depict the progression of fibrosis in patients with no or minimal fibrosis, as determined using FIB-4 ( C ) and APRI ( D ) scores derived from clinical parameters at the time of liver biopsy and at 3-year follow-up. P values indicate significant differences in fibrosis scores at 3 years. ( E ) Schematic shows our proposed model for GIV’s role in fibrogenic signalling in HSCs during liver fibrosis. Top to bottom: fibrogenic injuries of various kinds result in the activation of diverse classes of receptors that trigger upregulation of GIV in HSCs. Increased GIV triggers transformation of quiescent HSCs into activated myofibroblasts by modulating two key signalling pathways: (1) the profibrotic PI3K-Akt pathway and (2) the antifibrotic cAMP-PKA pathway. In quiescent HSCs low levels of GIV expression generate a net antifibrogenic signalling programme characterized by low Akt activity and impaired activation of Gαi with resultant high levels of cAMP. In activated HSCs, high levels of GIV expression generate a net profibrogenic signalling programme characterized by high Akt activity and increased activation of Gαi with resultant low levels of cAMP. Low GIV expression maintains HSCs in quiescent state, triggers apoptosis and suppresses collagen production in the normal liver, whereas high GIV expression enhances HSC migration, proliferation and survival, and triggers collagen production, thereby leading to liver fibrosis. n =number of patients. Error bars represent mean±s.d. Statistical significance was assessed with two-tailed Student’s t -test. Full size image Here we define GIV as a central hub within the fibrogenic signalling network downstream of multiple receptors. By virtue of its ability to activate trimeric G protein Gi, GIV simultaneously modulates pro- and antifibrotic pathways that function antagonistically to balance collagen synthesis and its removal in a delicate equilibrium. Our results provide detailed mechanistic insights into how GIV triggers HSC activation and supports the model outlined in Fig. 9E . In response to a variety of chronic injuries, diverse classes of fibrogenic receptors are activated, which triggers an upregulation of GIV mRNA, translation of GIV protein and its activation in HSCs. Increased expression of GIV and activation of its GEF function enhances PI3K-Akt and SMAD signals and blunts cAMP accumulation, both via activation of Gαi. These upstream events trigger subsequent tiers of signals along the pro- and antifibrogenic pathways (see Fig. 8 ), skewing the entire network towards an overall profibrotic signalling programme that favours fibrogenesis. Consequently, several phenotypes (migration, proliferation, actin remodelling, survival/antiapoptosis and collagen production) that are critical not only for transdifferentiation of HSCs to an active state but also for a sustained increase in the abundance of activated HSCs in the liver during progressive liver injury, eventually leading to liver fibrosis. Depletion of GIV, or targeted inhibition of its GEF function, reverses the profibrogenic programme in HSCs, that is, suppresses Akt activity and increases cellular cAMP, thereby 'resetting' the balance to an antifibrogenic programme, as exists in the normal liver. We conclude that GIV is a key transducer of signals downstream of multiple classes of fibrogenic receptors that trigger liver fibrosis. Of the many receptors that utilize GIV to transduce profibrotic signals, we found that the fibrogenic RTK PDGFRβ directly binds and phosphorylates GIV. This is in keeping with our previous work on the prototype RTK, EGFR, in which we defined how GIV serves as a signalling platform that links ligand-activated RTKs to G protein signalling. Although the other major profibrotic receptor, that is, TGFβR also requires GIV’s GEF function to enhance Akt and SMAD signals and collagen synthesis, surprisingly, we could not identify a direct link (neither binding nor phosphoregulation) between them. As TGFβ and PDGF pathways crosstalk [41] , [42] , [43] , we hypothesize that GIV and its GEF function may enhance Akt signals in response to TGFβ indirectly via activation of the PDGFR pathway. Similarly, as the PI3K-Akt pathway can potentiate fibrogenic SMAD signals in cells responding to TGFβ [44] , it is possible that GIV and its GEF function enhance SMAD signals via activation of Akt. We demonstrate that GPCRs, such as CCRs, also require GIV’s GEF function for enhancement of Akt activity when stimulated with RANTES. We previously demonstrated that GPCRs (for example, LPAR1 and f-Met-Leu-Pro-R) require GIV and its GEF function for PI3K-Akt signalling and chemotaxis [16] , [19] , [45] , and that they can trigger tyrosine phosphorylation and activation of GIV via activation of Src-family of non-RTKs [17] . We conclude that CCRs modulate pro- and antifibrogenic signals via activation of GIV. Finally, we also provide evidence that TLR4, a receptor that is unique to fibrosis in the liver, also requires GIV’s GEF function to enhance Akt signals when stimulated with LPS. Our findings are consistent with data showing that TLR4 requires activation of the PI3K-Akt pathway for enhancement of TGFβ-SMAD signalling [46] , [47] , and that cirrhosis-predictive single-nucleotide polymorphisms of TLR4 are functionally linked to genes of the PI3K-Akt pathway [48] . We conclude that TLR4 activates Akt via GIV, and results shown here provide the first evidence for how GIV may shape the innate immune response by modulating signalling networks initiated by members of the interleukin-1/TLR superfamily. As KCs are the main target of LPS in the liver [49] , and these cells also upregulated GIV mRNA after injury, it is possible that the TLR4-GIV-Akt pathway also helps to activate KCs during liver fibrosis. Besides demonstrating that multiple fibrogenic receptors converge upon GIV, we demonstrate that subsequent activation of Gαi by GIV modulates two functionally antagonistic signalling events (see Fig. 8 ): (a) activation of the profibrotic PI3K-Akt signals that potentiate TGFβ-SMAD signals and inhibit FoxO1 and (b) inhibition of cAMP production, which suppresses the PKA-pCREB pathway, thereby generating an overall profibrotic signalling programme that favours fibrosis. As the PI3K-Akt pathway is strongly implicated in studies of fibrogenic diseases in other organ systems (skin, cardiac, pulmonary (reviewed in ref. 50 )), and the cAMP pathway is a well-accepted antifibrotic pathway in various other models of fibrogenesis (cardiac [51] , pulmonary [42] , kidney [44] and skin [26] ), and fibrosis in all organs share common receptors/pathways defined here (that is, TGF-β1 and PDGF [52] ), we speculate that GIV may also serve as a key mediator in fibrogenic diseases of other organs. The other important finding is the invariable upregulation of GIV mRNA and expression of GIV protein after several forms of chronic liver injury, in both humans and mice. Although here we focused on upregulation of GIV in HSCs, it is noteworthy that other cells such as ECs and KCs that also contribute to liver fibrosis by promoting sustained activation of HSCs [53] showed significant upregulation of GIV after injury. This was not unexpected because GIV is known to be expressed in vascular endothelial cells [15] and we previously showed that GIV is required for macrophage chemotaxis [19] . As in the case of HSCs, activation and secretion of cytokines and chemokines by KCs is antagonistically balanced by the PI3K-Akt [7] and the cAMP-pCREB pathways [54] . As GIV modulates those two signalling pathways in HSCs, we suspect that GIV’s role in liver fibrosis is not limited to activation of HSCs but extends also to activation of KCs, all via common signal transduction mechanisms we outline here. As for mechanism(s) of GIV upregulation, our results indicate that its expression may be regulated at multiple steps. For example, quiescent HSCs have low levels GIV mRNA but no protein is translated, indicating that protein translation is repressed or protein half-life is short in these cells. However, in activated HSCs, high levels of GIV mRNA and full-length protein are seen, indicating that transcriptional induction and/or RNA and/or protein stabilization are responsible for such upregulation. We have recently defined STAT3 as a key transcription factor responsible for upregulation of GIV in response to wounding and during cancer progression [22] . Because STAT3 has been widely implicated in perpetuating inflammation/injury response in the liver [55] , and liver fibrosis has been linked to wound healing [23] , it is possible that STAT3 upregulates GIV after liver injury, thereby linking inflammation to fibrogenesis. Regardless of the mechanism(s) involved, we found that sustained upregulation of GIV is restricted to some forms of injuries, not others: upregulation occurs in all forms of chronic fibrogenic injuries but not in acute injuries that heal without fibrosis. These results indicate that GIV is not merely a component of an acute-phase response in the injured liver, instead, increased expression of GIV during acute injuries may signal a potential for progression to chronicity and fibrosis. With regard to the clinical relevance of our findings, we provide evidence that GIV could serve both as a therapeutic target against and a biomarker for prognosticating liver fibrosis. Our findings in HSCs expressing the GEF-deficient GIV-FA demonstrate that selective inhibition of the GIV:Gαi interface by a single point mutation is sufficient to alter a multitude of signals and inhibit various phenotypes that are required for sustained activation of HSCs. On the basis of these we conclude that the GIV:Gαi interface is an effective and specific target, which is also sensitive to disruption. Furthermore, since accumulation of cellular cAMP can reverse fibrosis [13] , and accumulation of cAMP is one of the direct consequences of inhibiting GIV’s GEF function, we anticipate that antagonists targeting the GIV:Gαi interface will not only halt but also cause regression of fibrosis by reinstating antifibrotic signalling. On the basis of our findings that GIV’s GEF function is utilized by multiple receptors, inhibiting the GIV:Gαi interface constitutes a novel strategy for externally manipulating multiple fibrogenic receptors via a single target. As full-length GIV is not expressed in the normal liver, and the majority of cells in the liver (that is, hepatocytes) do not express GIV even after injury, inhibition of GIV is likely to have fewer off-target effects on major metabolic functions of the liver. We conclude that small molecules against the GIV:Gαi interface have the potential of being both selective and broad—that is, selectively inhibit GIV-dependent profibrotic signalling in cells that express full-length GIV, yet broadly downstream of multiple receptors. With regard to the prognostic potential of GIV, we provide proof-of-concept that detection of GIV in formalin-fixed paraffin embedded (FFPE) liver biopsies early during the course of chronic HCV infection (when significant fibrosis is yet to occur) may predict rapid progression to advanced fibrosis. On the basis of the fact that GIV expression in HSCs precedes collagen synthesis and onset of liver fibrosis, GIV fits the definition of an ideal prognosticator that identifies at-risk patients even at early stages when minimal or no fibrosis is detected with IHC. In addition, our IHC results show that full-length GIV is detected easily and reproducibly with three different CT antibodies, and that a simple binary system of scoring (that is, presence or absence of GIV) is sufficient to distinguish at-risk individuals from others without the need for cumbersome and subjective scoring algorithms. Despite the potential significance of our findings, limitations of this and any future studies on this topic includes the frequent occurrence of sampling error in liver biopsies, despite the fact that individual biopsies meet the histologic criteria for adequacy. To circumvent this limitation, here we used two different clinical scoring methods to monitor the progression of fibrosis, FIB-4 and APRI; each score is derived from multiple clinical parameters. We found that both scores concurrently classified the patients into two groups—non-progressors (fibrosis stages F0=no fibrosis; F1=portal fibrosis without bridges; F2=portal fibrosis with rare bridges) and progressors (fibrosis stages F3=numerous bridges without cirrhosis; F4=cirrhosis). Our results indicate that expression of GIV in HSCs using IHC was associated with progression of fibrosis to significant levels within 3 years. We conclude that GIV may serve as a prognostication biomarker for clinical use to identify those patients with chronic liver injury that are at highest risk for progressive fibrosis. As growing evidence suggests that activated HSCs drive primary liver and biliary cancer progression [56] , and as GIV is a bona fide prometastatic protein that imparts aggressiveness to multiple cancers [22] , [57] , it is possible that levels of expression of GIV in HSCs correlate/predict progression to liver cancer. Further studies on larger cohorts of patients are required to evaluate whether GIV expression in liver biopsies independently predicts liver cirrhosis and/or progression to cancer. In conclusion, here we have defined GIV as a novel signalling hub at the centre of the complex multireceptor signalling system that drives liver fibrosis. Our findings set a new paradigm in which a single multidomain signal transducer centrally integrates and broadly shapes the entire fibrogenic network. As a promising therapeutic target that can serve as a biomarker to predict the risk of fibrosis, GIV presents an opportunity for the practice of personalized medicine in patients with fibrogenic diseases of the liver. Reagents and antibodies Unless otherwise indicated, all reagents were of analytical grade and obtained from Sigma-Aldrich. Cell culture media were purchased from Invitrogen. PDGF (Invitrogen), TGFβ1 (Invitrogen), RANTES (R&D Systems) and LPS-E Coli 055:B5 (Sigma) were obtained commercially. BrdU was obtained from Sigma-Aldrich. Recombinant and PDGFRβ was purchased from Cell Signaling. All restriction endonucleases and Escherichia coli strain DH5α were purchased from New England Biolabs. E. coli strain BL21 (DE3), oligofectamine and phalloidin-Texas Red were purchased from Invitrogen. 4',6-Diamidino-2-phenylindole (DAPI) was purchased from Molecular Probes (Invitrogen). Genejuice transfection reagent was obtained from Novagen (EMD Millipore) and PfuUltra DNA polymerase was purchased from Stratagene. Silencer Negative Control scrambled (Scr) siRNA was purchased from Ambion and a previously validated [32] GIV siRNA sequence was custom-ordered from Dharmacon. Goat anti-rabbit and goat anti-mouse Alexa Fluor 680 or IRDye 800 F(ab′) 2 used for Odyssey Infrared Imaging were from Li-Cor Biosciences. Antibodies used in this work include rabbit polyclonal antibodies (pAbs) against Gαi3 (M-14) and pan-Gβ (Santa Cruz Biotechnology), phospho-Akt Ser 473, phospho-ERK 1/2, phospho-SMAD 2 and phospho-CREB (Cell Signaling) and phospho-Histone H3 (Abcam). Mouse monoclonal antibodies (mAbs) against hexahistidine (His), FLAG (M2), actin and α-tubulin (Sigma-Aldrich), SMAD 2/3, phospho-PDGFRβ-Tyr716 and GFP (Santa Cruz Biotechnology), BrdU (BD Biosciences), PDGFRβ (Biolegend), α-SMA (DAKO), control IgG (Bio-Rad Laboratories) and anti-active Caspase 3 (Abcam) were obtained commercially. Several anti-GIV antibodies were used in this work. For immunoblotting, we used rabbit anti-GIV coiled-coil (GIVcc; Millipore) and GIV-CT Abs (Santa Cruz Biotechnology). Coiled-coil antibody detects most isoforms of GIV, whereas CT Ab detects exclusively the full-length isoform of GIV that contains the domains required for GIV’s function as a signal transducer. For immunofluorescence we used rabbit monoclonal anti-GIV-CT (Spring Bioscience) and anti-GIV-CT mAb (Millipore). Three different Anti-GIV-CT Abs were used for IHC detection of GIV (Santa Cruz Biotechnology, IBL America and Spring Bioscience). All these CT antibodies were raised against the last 18 amino acids of the C terminus and were validated in immunoblot assays based on their ability to specifically detect the full-length GIV isoform. Anti-Tyr1764-GIV Ab was developed by Spring Bioscience using a proprietary platform for the generation of Rabbit mAb using a peptide encompassing pY1764. It is a diagnostic grade antibody jointly developed by our group, Ventana/Roche and Spring Biosciences and extensively validated in multiple assays before being used in this project. Anti-Ser1614-GIV was commercially obtained from IBL America and was previously validated by the Takahashi group [32] . Anti-Gαi3:GTP (6-F12) was a gift from Dr Graeme Milligan [58] . Plasmid constructs, mutagenesis and protein expression Cloning of Gαi3 into pGEX-4T-1 (GST-Gαi3), GIV-CT (aa 1,660–1,870) into pET28b (His-GIV-CT) and RNA interference-resistant (siRNA rest) GIV was generated by silent mutations [32] and cloned into p3XFLAG-CMV-14 plasmid (GIV-FLAG) as described previously [16] , [19] , [26] , [45] . His-PCT (Podocalyxin Tail) was a gift from Dr Farquhar MG [59] . GIV mutants were generated using QuickChange II (Stratagene) and specific primers (sequence available upon request) following the manufacturer’s instructions. All constructs were checked by DNA sequencing. GST, GST-Gαi3, His-GIV-CT and His-PCT fusion constructs were expressed in E. coli strain BL21 (DE3) (Invitrogen) and purified as described previously [16] , [19] , [26] . Bacterial cultures were induced overnight at 25 °C with 1 mM isopropyl β- D -1-thiogalactopyranoside. Pelleted bacteria from 1 l of culture were re-suspended in 10 ml GST-lysis buffer [25 mM Tris-HCl, pH 7.5, 20 mM NaCl, 1 mM EDTA, 20% (v:v) glycerol, 1% (v:v) Triton X-100, 2X protease inhibitor cocktail (Complete EDTA-free, Roche Diagnostics)] or His-lysis buffer [50 mM NaH 2 PO 4 , pH 7.4, 300 mM NaCl, 10 mM imidazole, 1% (v:v) Triton X-100, 2X protease inhibitor cocktail (Complete EDTA-free, Roche Diagnostics)] for GST or His-fused proteins, respectively. After sonication (3 × 30 s), lysates were centrifuged at 12,000 g at 4 °C for 20 min. Solubilized proteins were affinity-purified on glutathione-Sepharose 4B beads (GE Healthcare) or HisPur Cobalt Resin (Pierce). Proteins were eluted, dialysed overnight against phosphate-buffered saline (PBS) and stored at −80 °C. Mice and fibrosis induction Expression of collagen type I time was studied using reporter Col-GFP mice (pCol9GFP-HS4,5 transgene) [30] . For all other experiments, 8- to 12-week-old male C57BL/6 mice (Jackson Laboratories) underwent BDL surgery or administration of CCl 4 exactly as described previously [7] . Sham operation was performed similarly, except that the bile duct was not ligated. Animals were killed 5 or 21 days after BDL. CCl 4 (Sigma-Aldrich; diluted 1:3 in corn oil) or vehicle (corn oil) was administered via intraperitoneal route at a dose of 0.5 μl per g body weight, twice per week, for a total of 12 injections. Animals received humane care according to NIH recommendations outlined in the ‘Guide for the Care and Use of Laboratory Animals.’ All animal experiments and cell isolation studies were approved by the UCSD Institutional Animal Care and Use Committees. Isolation and culture of liver cell fractions from mice Liver cells of 8- to 12-week-old male C57BL/6 mice (Jackson Laboratories) were fractionated into hepatocytes, KCs, endothelial cells and HSCs as previously described [60] . Perfusion of mouse livers was followed by three-layer discontinuous density gradient centrifugation with 8.2 and 14.5% Nycodenz (Accurate Chemical and Scientific Corporation). KC or endothelial cell fractions were then selected positively using magnetic cell sorting using anti-CD11b antibody or antiliver sinusoidal endothelial cell antibody, respectively (Miltenyi Biotech). The HSC fraction was purified by negative selection for KCs and endothelial cells using magnetic cell sorting with respective antibodies. These cell fractions were homogenized immediately for RNA extraction. The purity levels of hepatocytes, HSCs and ECs were examined using phase-contrast microscopy, ultraviolet (UV)-excited autofluorescence (HSC) and uptake of diacetylated low-density lipoprotein (EC). The purity of KC was demonstrated by functional analysis by means of phagocytosis of 1-μm latex beads. The purity of each cell type was as follows: hepatocytes, greater than 97%; EC, greater than 98%; KC, greater than 95%; and HSC, greater than 96%. When we isolated HSCs for use in various assays throughout the manuscript, purity was confirmed as >98% by immunostaining with anti-desmin antibody. HSCs were cultured on uncoated plastic tissue culture dishes/coverslips in DMEM containing 10% fetal bovine serum (FBS) and used as primary cultures only. RNA isolation and quantitative PCR (qPCR) Total RNA was isolated using an RNeasy kit (QIAGEN) as per the manufacturer’s protocol. First-strand cDNA was synthesized using Superscript II reverse transcriptase (Invitrogen), followed by ribonuclease H treatment (Invitrogen) before performing quantitative real-time PCR. Reactions omitting reverse transcriptase were performed in each experiment as negative controls. Reactions were then run on a real-time PCR system (ABI StepOnePlus; Applied Biosystems). Gene expression was detected with SYBR green (Invitrogen), and relative gene expression was determined by normalizing to GAPDH using the ΔΔ T method. Primers used in this work were designed targeting the last two exons of GIV such that they exclusively detect all known full-length isoforms of GIV using Invitrogen’s Oligo Perfec Designer and evaluated with NetPrimer from Premierbiosoft [26] . The sequences of primers used in this work are included in Supplementary Table 1 . Patient samples Human liver samples used for GIV mRNA analysis were collected at the Mount Sinai Hospital. Cirrhosis samples were collected from HCV-infected patients undergoing surgical resection or liver transplantation for hepatocellular carcinoma. Normal liver tissue was collected from patients receiving hepatic resections for non-tumoral diseases, including hepatic adenoma and focal nodula hyperplasia. Liver samples were snap-frozen, and RNA was extracted, DNase-treated, reverse transcribed and analysed using quantitative real-time PCR as described above. Liver biopsy specimens used in this work for IHC were obtained from 21 patients undergoing percutaneous liver biopsies from year 2009 to 2010 at the VA San Diego Healthcare System. Biopsies were performed using a standard Jamshidi aspiration needle and samples were formalin-fixed immediately and embedded in paraffin. Adequacy of the biopsy specimen was established by the presence of at least six to eight portal triads. In addition, seven specimens of the normal liver were obtained from autopsies performed by the County of San Diego. All tissues used in this work were collected after IRB approval (Project no. 04-0056 0001 05 ME X and 101264) and with informed patient consent. As for limitations of this study, although the biopsies were carried out according to standard clinical practice and met current criteria for liver biopsy sampling, it is well known that sampling error can occur with liver biopsies despite meeting histologic criteria for individual biopsies. Despite the fact that sampling error is possible, this remains the ‘gold standard’ for determination of liver histology. Immunohistochemistry GIV IHC assays were developed and performed on a BenchMark XT automated slide stainer (Ventana Medical Systems Inc.). FFPE samples (4-μm section) were deparaffinized, pretreated for antigen retrieval and followed by inactivation of endogenous peroxidase. Specimens were incubated with anti-GIV rabbit monoclonal (Ventana Medical Systems Inc.) or polyclonal (IBL, Santa Cruz Biotechnology) antibodies (10 μg ml −1 ) for 16 min at 37 °C and the immunolocalized proteins were visualized using the OptiView DAB IHC Detection kit. Following detection, all samples were counterstained with the Hematoxylin II and Bluing Reagent. There was 100% concordance between all antibodies tested. Semithin immunofluorescence Liver specimens were fixed with 4% paraformaldehyde for 4 h at 4 °C, and cryoprotected and frozen in liquid nitrogen. Semithin sections (0.5 μm) were cut with a Leica Ultracut UCT microtome equipped with a FCS cryoattachment at −100 °C. Frozen sections were washed with PBS (3 × ), washed with 0.15% glycine (2 × ) and incubated 20 min in blocking buffer (5% normal goat serum, 2% fish skin gelatin and 2 mg ml −1 of bovine serum albumin (BSA) in PBS), 2 h in primary antibodies and 45 min in secondary antibodies. Dilutions of antibodies used were as follows: Mouse anti-GIV-CT (1:30), GFP (1:50); α-SMA (1:200); DAPI (1:1,000) and secondary goat anti-mouse (594), goat anti-rabbit (488) and goat anti-rabbit (635) Alexa-conjugated antibodies (1:250). Sections were imaged on a Leica SPE confocal microscope using a × 63 oil objective using 488, 561, 633 and 405 laser lines for excitation. The settings were optimized and the final images scanned with line-averaging of 3. All images were processed using the Image J software (NIH) and assembled for presentation using Photoshop and Illustrator softwares (Adobe). Whole-cell Immunofluorescence Lx2 cells were fixed with 3% paraformaldehyde in PBS for 25 min at room temperature, treated with 0.1 M glycine for 10 min and subsequently blocked/permeabilized with PBS containing 3% BSA and 0.2% Triton X-100 for 30 min at room temperature. Primary and secondary antibodies were incubated for 1 h at room temperature in PBS containing 3% BSA and 0.2% Triton X-100. Cells were imaged on a Leica SPE confocal microscope using a × 63 oil objective using 488, 561 and 405 laser lines for excitation. The settings were optimized and the final images scanned with line-averaging of 3. Dilutions of antibodies used were as follows: GIVcc (1:150); GM130 (1:150); phospho-GIV (Tyr1764; 1:500); phospho-PDGFRβ (1:50); PDGFRβ (1:100); mouse anti-GIV-CT (1:100); Phalloidin (1:1,000); DAPI (1:2,000); secondary goat anti-rabbit (594) and goat anti-mouse (488) Alexa-conjugated antibodies (1:500); anti-phospho-Histone H3 (Ser28) (1:150), anti-BrdU (1:10), SMAD 2/3 (1:100), phospho-CREB (1:250), FoxO1 (1:100) and anti-active Caspase 3 (1:200). All images were processed using the Image J software (NIH) and assembled for presentation using Photoshop and Illustrator softwares (Adobe). For assays investigating nuclear localization of transcription factors, % cells with nuclear localization was quantified by counting any nuclear staining as presence of transcription factor in the nucleus, and used that as a basis for a binary system (that is, cells with or without nuclear localization of transcription factor). Approximately 200–400 cells per condition were counted from three independent experiments. Cell Culture, transfection, lysis and quantitative immunoblotting The Lx2 human HSC line was obtained from Scott Friedman (Mount Sinai, NY) and were cultured in DMEM media containing 2% FBS according to the previously published guidelines [31] . Transfection, lysis and immunoblotting were carried out exactly as described before [19] , [26] , [61] . Lx2 cells were transfected using Genejuice (Novagen) for DNA plasmids and Oligofectamine (Invitrogen) for siRNA oligos following the manufacturers’ protocols. For adenovirus infection, cells were incubated with the respective viruses at 50 multiplicity of infection for 5 h. Afterwards, the medium was replaced and cells were maintained for 2–3 days. For assays involving serum starvation, serum concentration was reduced to 0% overnight and for serum reduced treatment 0.2% FBS was used. Whole-cell lysates were prepared after washing cells with cold PBS before resuspending and boiling them in sample buffer. Lysates used as a source of proteins in immunoprecipitation or pull-down assays were prepared by resuspending cells in lysis buffer (20 mM HEPES, pH 7.2, 5 mM Mg-acetate, 125 mM K-acetate, 0.4% Triton X-100, 1 mM DTT, supplemented with sodium orthovanadate (500 μM), phosphatase (Sigma) and protease (Roche) inhibitor cocktails)), after which they were passed through a 28G needle at 4 °C, and cleared (10,000 g for 10 min) before being used in subsequent experiments. For immunoblotting, protein samples were separated using SDS–PAGE and transferred to polyvinylidene difluoride membranes (Millipore). Membranes were blocked with PBS supplemented with 5% nonfat milk (or with 5% BSA when probing for phosphorylated proteins) before incubation with primary antibodies. Infrared imaging with two-colour detection and quantification were performed using a Li-Cor Odyssey imaging system. Dilution of primary antibodies were used as follows: Anti-His 1:1,000; anti-FLAG 1:500; anti-GIV-CT 1:500; anti-phospho-GIV (Tyr1764) 1:500; anti-phospho-GIV (Ser1416) 1:500; anti-phospho-Akt 1:250; anti-Akt 1:500; anti-phospho-ERK 1/2 1:250; anti-Gαi3 1:333; anti-pan-Gβ 1:250; anti-α tubulin 1:2,000; anti-actin 1:1,000; anti-SMAD 2/3 1:250; anti-phospho-PDGFRβ 1:250; anti-PDGFRβ 1:250 and anti-phospho-CREB (1:1,000). All Odyssey images were processed using the Image J software (NIH) and assembled for presentation using Photoshop and Illustrator softwares (Adobe). Uncropped images of immunoblots are shown in Supplementary Figs 7–9 . Cell migration and proliferation assays Lx2 cells were transfected with control scrambled (Scr) siRNA or GIV siRNA for ~36 h. Monolayer cultures (100% confluent) were then scratch-wounded using a 20-μl pipette tip, and the cells were subsequently monitored using phase-contrast microscopy over the next 24 h. To quantify cell migration (expressed as percent of wound closure), images were analysed using the Image J software to calculate the difference between the wound area at 0 h and that at 24 h divided by the area at 0 h × 100. The proliferation rate of Lx2 cells was measured by phospho-Histone H3 (Ser28) (mitotic index) and BrdU incorporation (DNA replication in the S phase) as previously described [20] . For the mitotic index, cells were grown on coverslips for 24 h, and then fixed and analysed using confocal microscopy. For the BrdU uptake assay, Lx2 cells were grown on coverslips for 24 h and treated with 10 μM BrdU for 30 min. Cells were then fixed with 70% ethanol for 30 min at room temperature, washed with PBS (3 × ), treated with 2 M HCl for 20 min at room temperature, followed by 0.1 M Na 2 B 4 0 7 (pH 8.5) for 2 min at room temperature. Finally, coverslips were washed with PBS (3 × ) and analysed using confocal microscopy. For both phospho-Histone and BrdU assays, 400–600 cells from 10 randomly chosen fields were counted (DAPI-stained) from three independent experiments. Mitotic index was determined by dividing the number of positively stained cells/the total number of DAPI-stained nuclei × 100. Results are shown as mean±s.e.m. of 10 fields from three separate experiments. For the mitotic index in primary murine HSCs, cells were isolated from mouse liver and grown on coverslips for 16 h. Then, mHSCs were infected with GIV-WT or GIV-FA adenoviruses and 24 h later cells were starved or treated with PDGF-BB (20 ng ml −1 16 h) and the mitotic index was measured using confocal microscopy. Assays for measuring cellular apoptosis Three different approaches were used. Lx2 cells were grown on coverslips and either transfected with control scrambled (Scr) siRNA or GIV siRNA for 48 h or infected with GIV-WT or GIV-FA adenoviruses and 24 h later, cells were starved for another 24 h. To measure Caspase 3 cleavage, cells were fixed and stained with anti-active Caspase 3 Ab (1:200). Measurement of DNA fragmentation using the TUNEL assay was performed according to the protocol of In situ Cell Death Detection Kit, TMR red (Roche). A total of 100 cells from randomly chosen fields were counted (DAPI-stained) from three independent experiments. The percent of cells with either active Caspase 3 or fragmented DNA was determined by dividing the number of positively stained cells/the total number of DAPI-stained nuclei × 100. Expression of two bona fide pro- (Bax) and anti (Bcl-2)-apoptotic signalling intermediates was measured using qPCR. Generation of adenoviruses expressing GIV HA-tagged full-length human GIV-WT and GIV-F1685A (GIV-FA) resistant to siRNA against human and murine GIV were cloned into the pShuttle-CMV vector [62] . The resultant plasmid was linearized with PacI and transformed into electrocompetent AdEasier E.coli (Agilent) using a Gene Pulser Electroporator (Bio-Rad). Correctly recombined clones were chosen based on sequencing and restriction endonuclease analyses, linearized with PacI and transfected into Cre8 cells (a gift from Dr Ora Weisz, University of Pittsburgh). Adenoviral particles were amplified using HEK-293 cells and purification was performed using caesium chloride gradients [62] . In vitro pull-down assays and immunoprecipitation Purified GST-Gαi3, GST alone, His-GIV-CT or His-PCT were immobilized on either glutathione-Sepharose or HisPur Cobalt beads for 90 min at room temperature as described before [17] , [19] , [26] , [63] . Lx2 HSCs lysates or phosphorylated PDGFRβ (50 ng) proteins were added to each tube, and binding reactions were carried out for 4 h at 4 °C with constant tumbling in binding buffer (50 mM Tris–HCl (pH 7.4), 100 mM NaCl, 0.4% (v:v) Nonidet P-40, 10 mM MgCl 2 , 5 mM EDTA, 2 mM DTT, protease inhibitor mixture). Beads were washed (4 × ) with 1 ml of wash buffer (4.3 mM Na 2 HPO 4 , 1.4 mM KH 2 PO 4 (pH 7.4), 137 mM NaCl, 2.7 mM KCl, 0.1% (v:v) Tween 20, 10 mM MgCl 2 , 5 mM EDTA, , 2 mM DTT) and boiled in Laemmli’s sample buffer. When GST-Gαi3 was used in the assay, both binding buffer and washing buffer were supplemented with 30 μM GDP. For immunoprecipitation, cell lysates (~2 mg of protein) were incubated for 4 h at 4 °C with 2 μg anti-PDGFR mAb or pre-immune control mouse IgG. Protein G Sepharose beads (GE Healthcare) were added and incubated at 4 °C for an additional 60 min. Beads were washed and bound immune complexes were eluted by boiling in Laemmli’s sample buffer. For immunoprecipitation of active Gαi3, cell lysates were incubated for 1 h at 4 °C with the conformational Gαi3: GTP mouse antibody (1 μg) [58] or pre-immune control mouse IgG. Protein G Sepharose beads (GE Healthcare) were added and incubated at 4 °C for additional 45 min. Beads were washed and immune complexes were eluted by boiling in Laemmli’s sample buffer as previously described [59] , [61] , [62] . In vitro kinase assay In vitro kinase assays were performed using purified His-GIV-CT or His-PCT proteins (~5 μg) and commercially obtained PDGFRβ kinase (Cell Signaling). Reactions were started by addition of 1,000 μM ATP and were carried out at 25 °C for 60 min in 30 μl kinase buffer (60 mM Hepes (pH 7.5), 5 mM MgCl 2 , 5 mM MnCl 2 , 3 μM Na 3 OV 4 ). Reactions were stopped by addition of Laemmli’s sample buffer and by boiling. Measurement of cAMP Lx2 cells were transfected with GIV-WT or GIV-FA, serum-starved (0% FBS, 16 h) and incubated with isobutylmethylxanthine (200 μM, 20 min) followed by PDGF (20 ng ml −1 , 10 min) and Forskolin (10 μM, 10 min). Reactions were terminated by aspiration of media and addition of 150 μl of ice-cold TCA 7.5% (w/v). cAMP content in TCA extracts was determined by radioimmunoassay and normalized to protein (determined using a dyebinding protein assay (Bio-Rad)) [64] . Data are expressed as fold change over Forskolin stimulation. Data analysis and statistics All experiments were repeated at least three times, and results were presented either as one representative experiment or as average±s.d. Statistical significance was assessed with two-tailed Student’s t -test. How to cite this article: Lopez-Sanchez, I. et al. GIV/Girdin is a central hub for profibrogenic signalling networks during liver fibrosis. Nat. Commun. 5:4451 doi: 10.1038/ncomms5451 (2014).